Host ICAMs play a role in cell invasion byMycobacterium tuberculosisandPlasmodium falciparum Intercellular adhesion molecules (ICAMs) belong to the immunoglobulin superfamily and participate in diverse cellular processes including host–pathogen interactions. ICAM-1 is expressed on various cell types including macrophages, whereas ICAM-4 is restricted to red blood cells. Here we report the identification of an 11-kDa synthetic protein, M5, that binds to human ICAM-1 and ICAM-4, as shown by in vitro interaction studies, surface plasmon resonance and immunolocalization. M5 greatly inhibits the invasion of macrophages and erythrocytes by Mycobacterium tuberculosis and Plasmodium falciparum , respectively. Pharmacological and siRNA-mediated inhibition of ICAM-1 expression also results in reduced M. tuberculosis invasion of macrophages. ICAM-4 binds to P. falciparum merozoites, and the addition of recombinant ICAM-4 to parasite cultures blocks invasion of erythrocytes by newly released merozoites. Our results indicate that ICAM-1 and ICAM-4 play roles in host cell invasion by M. tuberculosis and P. falciparum , respectively, either as receptors or as crucial accessory molecules. Any discourse on the scenario of infectious diseases, especially in the developing world, invariably includes tuberculosis (TB) and malaria, reiterating their impact on the current global public health situation. WHO (World Health Organization) studies indicate almost 8.6 million new cases and 1.3 million TB deaths in 2012 (ref. 1 ). TB is caused by Mycobacterium tuberculosis (Mtb) that primarily, although not exclusively, invades lung phagocytic cells such as macrophages, neutrophils, monocytes and dendritic cells (DCs). The incidence of malaria is equally staggering, at 207 million cases, with 627,000 deaths reported by WHO for the year 2012 (ref. 2 ). One of the main reasons for such high number of infections is the emergence of resistance to the currently available drugs, as well as a severe paucity of new drugs that can be added to the chemotherapy regimen. Rifampicin and Artemisinin—recommended components of first-line therapy against these diseases [3] , [4] —were discovered in 1963 and 1973, respectively. There is thus an urgent need to identify new drug targets and develop new drugs against these pathogens. Mtb and P. falciparum use multiple mechanisms to gain entry into their respective host cells. Like many other bacteria, Mtb utilizes complement receptors (CRs) and Toll-like receptors (TLRs) for invading phagocytic cells. Other receptors involved in Mtb internalization include mannose receptors [5] , surfactant protein A (Sp-A) and Sp-A receptors [6] , CD14 (ref. 7 ), scavenger receptors [8] and DC-specific intercellular adhesion molecule (ICAM)-3 grabbing nonintegrin [9] . More recent reports implicate cell surface CCR5 in Mtb pathogenesis albeit not as a direct receptor, but rather as a signal transducer involved in disease progression [10] . Another study has identified mycobacterial cell wall-associated Rv3083 as an agonist of TLR2 in order to activate macrophages [11] . Despite the expanding knowledge of roles of such potential receptors, there has been little success in using them to develop new therapeutics or immune modulators for treating Mtb infection. In the context of malaria, the invasion of red blood cells (RBCs) begins with an initial interaction of P. falciparum merozoites with the RBC surface, followed by re-orientation that allows the apical end of the merozoite to interact with the host cell membrane. The RBC surface molecules currently characterized as receptors for this pathogen include members of the glycophorin family [12] , [13] , CR1 (ref. 14 ), the recently identified Basigin [15] and Semaphorin 7A [16] . While receptor–ligand interactions between glycophorin members and CR1 have been characterized as ‘nonessential’ across many P. falciparum strains, Basigin, thus far, is the only blood-group antigen that has been validated as ‘essential’ for blood-stage growth of the parasite irrespective of its resistance status [15] . As yet, for several known parasite ligands, their receptors on RBC surface remain unknown. ICAMs (ICAM-1 to ICAM-5) are members of the Ig superfamily and are structurally similar, consisting of varying number of extracellular Ig domains stabilized by disulfide bonds, a transmembrane region and a short cytoplasmic tail [17] . Most ICAMs are expressed on a variety of cell types such as endothelial and epithelial cells, lymphocytes, monocytes, eosinophils, and ancestral haemopoietic cells—except ICAM-4 (Landstein–Weiner blood-group antigen) that is found exclusively on RBCs. Although the level of ICAM-4 expression on erythrocyte surface decreases as they progress through various stages of reticulocyte maturation, it is expressed to at least easily detectable levels in mature erythrocytes [18] , [19] . Among the various ICAMs, ICAM-1 (CD54) was the first to be described and studied extensively [20] . ICAM-1 serves as a pathogen receptor for the major group of Human Rhinoviruses [21] , [22] as well as for Coxsackievirus VA21 (ref. 23 ). The progression of West Nile virus across the blood brain barrier has also been attributed to an increased expression of ICAM-1 (ref. 24 ). Ever since, the role of ICAM-1 in the context of host–pathogen interactions continues to be an area of active research. HIV-1, for example, acquires integrins including LFA-1 during budding, and the integrin-bound viral particles interact with ICAM-1 and show an increased infectivity in nonsusceptible host cells [25] . In P. falciparum infection, ICAM-1 and CD36 have been shown to interact with infected erythrocytes and contribute to specific pathologies of cerebral malaria [26] . In the present study, using ‘codon-shuffled’ synthetic libraries [27] , [28] , we identify an 84 amino-acid (aa)-long de novo protein, M5, that binds both ICAM-1 and ICAM-4 potently. Addition of M5 during Mtb infection of THP-1 cells as well as murine peritoneal macrophages reduce Mtb invasion significantly. The use of a known ICAM-1 expression inhibitor, and ICAM-1 silencing by short interfering RNA (siRNA), results in a drastic reduction in Mtb infection, confirming the role of ICAM-1 during the infection process. We also determine the effect of M5 on the P. falciparum invasion of human RBCs. Addition of M5 significantly blocks P. falciparum invasion, uniformly across drug-susceptible (3D7) and drug-resistant parasite strains (Dd2, HB3 and MCamp). Together, these results are indicative of a receptor-like role of ICAMs for host cell invasion by two important intracellular pathogens, Mtb and P. falciparum , and also unveil alternative drug targets for the development of new inhibitors based on the interactions reported here. ICAM-1 is involved in Mtb host–pathogen interactions To identify novel host factors involved in Mtb invasion of human cells, a library-based protein–protein interaction analysis was performed using the Bacteriomatch two-hybrid system. An Mtb H37Rv genomic DNA library cloned in pBTnn vector [29] , a modified plasmid from the two-hybrid pBT vector, was screened with a human lung cDNA library cloned in the pTRG vector, to find interacting partners. On the basis of a blue–white selection, two colonies positive for interaction(s) were selected and sequenced. Blast analysis identified that both pairs of interacting partners had a 271-aa-long fragment of ICAM-1 that comprises a portion of the extracellular region (D3D5 domains), transmembrane region as well as the cytoplasmic tail (hereafter referred to as ICAM-1 271 ) in pTRG and two different mycobacterial metabolic proteins: a 128-aa-long C-terminal region of acetolactate synthase (large subunit), IlvB2 and an 83-aa-long C-terminal region of 3-hydroxybutyryl-CoA dehydrogenase, a known secretory protein (Rv1715 and fadB3; Fig. 1a ) in pBTnn. The sequences were analysed with NCBI BLAST and their theoretical protein parameters were computed using the ExPASy ProtParam tool ( Fig. 1b ). Sequences of the proteins are provided in Supplementary Figs 1a,b and 2 . The interactions were confirmed over repeated rounds of re-transformation and segregation of plasmids. 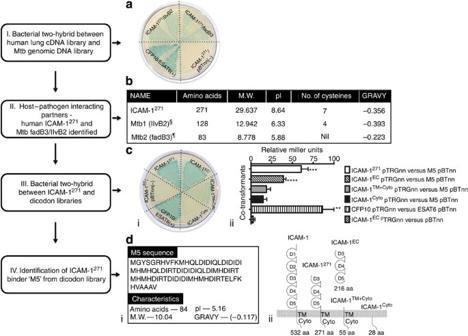Figure 1: Identification ofde novoprotein binder to ICAM-1. (a) X-gal indicator plate of bacterial two-hybrid experiment between human lung cDNA and Mtb genomic DNA libraries. All streaks are labelled to represent genes cloned in pTRG/pBTnn. ICAM-1271pTRG/empty pBTnn is the negative control; CFP10pTRGnn/ESAT6pBTnn is the positive control. (b) Protein parameters highlighting length, molecular weight (MW), isoelectric point (pI), number of cysteines and grand average of hydropathicity (GRAVY) of the identified host–pathogen protein interactors. Sequences of the identified proteins are provided inSupplementary Figs 1 and 2. (c) Bacterial two-hybrid assay to identifyde novoprotein/peptide binder to ICAM-1271and its domains. (i) X-gal indicator plate. All streaks are labelled to represent genes cloned in pTRGnn/pBTnn. (ii) Liquid β-galactosidase assay to measure relative enzyme activity (M.U.) of co-transformant pairs. Relative Miller units: ICAM-1271pTRGnn versus M5pBTnn (60.49±4.255); ICAM-1ECpTRGnn versus M5pBTnn (39.02±1.583); ICAM-1TM+CytopTRGnn versus M5pBTnn (18.71±4.855); ICAM-1CytopTRGnn versus M5pBTnn (14.70±2.176); positive control—CFP10pTRGnn versus ESAT6pBTnn (86.10±6.949); negative control—ICAM-1ECpTRGnn versus empty pBTnn (2.779±1.014). The graph is the average of three independent assays and s.d. is represented by error bars. All values were tested for significance using a two-tailed unpaired Student’st-test with Welch’s correction. **P<0.01, ***P<0.001, ****P<0.0001. (d) (i) Amino-acid sequence of the identifiedde novoM5 polypeptide. Protparam tool from the ExPASy server (http://web.expasy.org/protparam/) was used to ascertain MW, pI and hydrophobicity of M5. (ii) Schematic showing a comparison of full-length ICAM-1 transmembrane protein (532 amino acids) with ICAM-1271and its various fragments: ICAM-1271(271 amino acids), ICAM-1EC(216 amino acids), ICAM-1TM+Cyto(55 amino acids) and ICAM-1Cyto(28 amino acids).§IlvB2—N-terminal putative acetolactate synthase large subunit;¶fadB3—C-terminal 3-hydroxybutyryl-CoA dehydrogenase; EC—extracellular; TM+Cyto—transmembrane+cytoplasmic tail; Cyto—cytoplasmic tail. Figure 1: Identification of de novo protein binder to ICAM-1. ( a ) X-gal indicator plate of bacterial two-hybrid experiment between human lung cDNA and Mtb genomic DNA libraries. All streaks are labelled to represent genes cloned in pTRG/pBTnn. ICAM-1 271 pTRG/empty pBTnn is the negative control; CFP10pTRGnn/ESAT6pBTnn is the positive control. ( b ) Protein parameters highlighting length, molecular weight (MW), isoelectric point (pI), number of cysteines and grand average of hydropathicity (GRAVY) of the identified host–pathogen protein interactors. Sequences of the identified proteins are provided in Supplementary Figs 1 and 2 . ( c ) Bacterial two-hybrid assay to identify de novo protein/peptide binder to ICAM-1 271 and its domains. (i) X-gal indicator plate. All streaks are labelled to represent genes cloned in pTRGnn/pBTnn. (ii) Liquid β-galactosidase assay to measure relative enzyme activity (M.U.) of co-transformant pairs. Relative Miller units: ICAM-1 271 pTRGnn versus M5pBTnn (60.49±4.255); ICAM-1 EC pTRGnn versus M5pBTnn (39.02±1.583); ICAM-1 TM+Cyto pTRGnn versus M5pBTnn (18.71±4.855); ICAM-1 Cyto pTRGnn versus M5pBTnn (14.70±2.176); positive control—CFP10pTRGnn versus ESAT6pBTnn (86.10±6.949); negative control—ICAM-1 EC pTRGnn versus empty pBTnn (2.779±1.014). The graph is the average of three independent assays and s.d. is represented by error bars. All values were tested for significance using a two-tailed unpaired Student’s t -test with Welch’s correction. ** P <0.01, *** P <0.001, **** P <0.0001. ( d ) (i) Amino-acid sequence of the identified de novo M5 polypeptide. Protparam tool from the ExPASy server ( http://web.expasy.org/protparam/ ) was used to ascertain MW, pI and hydrophobicity of M5. (ii) Schematic showing a comparison of full-length ICAM-1 transmembrane protein (532 amino acids) with ICAM-1 271 and its various fragments: ICAM-1 271 (271 amino acids), ICAM-1 EC (216 amino acids), ICAM-1 TM+Cyto (55 amino acids) and ICAM-1 Cyto (28 amino acids). § IlvB2—N-terminal putative acetolactate synthase large subunit; ¶ fadB3—C-terminal 3-hydroxybutyryl-CoA dehydrogenase; EC—extracellular; TM+Cyto—transmembrane+cytoplasmic tail; Cyto—cytoplasmic tail. Full size image M5 binds ICAM-1 and disrupts its dimerization Since ICAM-1 was identified as a possible host factor involved in Mtb host–pathogen interactions, we next screened a dicodon polypeptide synthetic library to identify potential de novo peptide/protein binders to ICAM-1 271 . Two-hybrid screening was performed with ICAM-1 271 cloned into pTRGnn plasmid and a dicodon shuffled polypeptide library cloned in pBTnn. A de novo , 84-aa-long protein, named M5 ( Fig. 1d , left) was identified after several rounds of segregation, re-cloning and re-transformations. We further tested the M5 interaction with different domains of ICAM-1: extracellular (ICAM-1 EC ), transmembrane (ICAM-1 TM+Cyto ) and cytoplasmic (ICAM-1 Cyto ) based on the structural information available for ICAM-1 (refs 30 , 31 ) ( Fig. 1c,d , right). As shown in Fig. 1c (left), interaction was observed between M5 and ICAM-1 271 as well as with ICAM-1 EC . However, no such interaction was observed between M5 and ICAM-1 Cyto . The strengths of these interactions were further corroborated by quantitative liquid β-galactosidase enzyme assays ( Fig. 1c , right). The well-studied interaction between two mycobacterial proteins, CFP10 and ESAT6, was used as a positive control [32] . On host leukocytes, ICAM-1 predominantly exists as a dimer, and it is in this form that it binds its natural ligands like LFA-1 and Mac-1. To study whether the bacterially expressed ICAM-1 271 or its fragments also exhibit dimerization, genes corresponding to ICAM-1 271 or its fragments were cloned into both pTRGnn and pBTnn vectors and interaction studies performed. ICAM-1 271 /ICAM-1 271 and ICAM-1 EC /ICAM-1 EC pairs showed significant interactions, while ICAM-1 TM+Cyto /ICAM-1 TM+Cyto displayed it to a lesser extent ( Fig. 2a , left). The dimeric interactions were subsequently quantified via a liquid β-galactosidase enzyme assay ( Fig. 2a , right). We next evaluated the effect of M5 on ICAM-1 dimerization using a bacterial three-hybrid system developed previously by us [33] . The system allowed us to transform the ‘blue’ two-hybrid R1 reporter strain carrying ICAM-1 271 pTRGnn and ICAM-1 271 pBTnn vectors, with a third compatible plasmid pMTSA-expressing M5 protein. The gene cloned in pMTSA vector was under the tight regulation of the arabinose-inducible pBAD promoter and the triple transformant clones were plated on X-gal indicator plates with and without L-arabinose. Expression of M5 in the presence of L-arabinose turned the ICAM-1 271 /ICAM-1 271 -expressing strain from blue to white, indicating that ICAM-1 dimerization was disrupted by M5 ( Fig. 2b ). Expression of the reporter lacZ was monitored over incremental L-arabinose concentrations ( Fig. 2c , left), and the increase in M5 induction ( Fig. 2c , right) corresponded with declining reporter enzyme activity confirming the disruption. 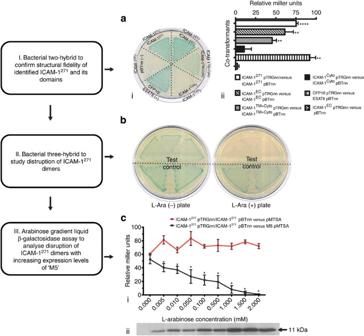Figure 2: Disruption of ICAM-1271dimerization by M5. (a) Bacterial two-hybrid assay to assess structural fidelity of ICAM-1271and its domains. (i) X-gal indicator plate. All streaks are labelled to represent genes cloned in pTRGnn/pBTnn. (ii) Liquid β-galactosidase assay to measure relative enzyme activity (M.U.) of co-transformant pairs: ICAM-1271pTRGnn versus ICAM-1271pBTnn (75.16±1.519); ICAM-1ECpTRGnn versus ICAM-1ECpBTnn (61.28±6.111); ICAM-1TM+CytopTRGnn versus ICAM-1TM+CytopBTnn (45.45±3.041); ICAM-1CytopTRGnn versus ICAM-1CytopBTnn (10.77±5.195); positive control—CFP10pTRGnn versus ESAT6pBTnn (92.19±4.195); negative control—ICAM-1ECpTRGnn versus empty pBTnn (2.249±1.189). The graph is the average of three independent assays and s.d. is represented by error bars. All values were tested for significance using a two-tailed unpairedt-test with Welch’s correction. **P<0.01, ****P<0.0001. (b) Bacterial three-hybrid X-Gal indicator plate (i) without L-Arabinose and (ii) with L-Arabinose.Test streaks:triple co-transformant containing ICAM-1271pTRGnn, ICAM-1271pBTnn and M5pMTSA;control streaks: triple co-transformant containing ICAM-1271pTRGnn, ICAM-1271pBTnn and empty pMTSA. (c) L-Arabinose gradient liquid β-galactosidase assay. (i) Relative β-galactosidase activity (M.U.) of the triple co-transformants ICAM-1271pTRGnn/ICAM-1271pBTnn versus empty pMTSA (red line) and ICAM-1271pTRGnn/ICAM-1271pBTnn versus M5pMTSA (black line), is plotted against a range of L-Arabinose concentrations. The graph is the average of three independent assays and s.d. is represented as error bars. Multiple unpairedt-tests to compare enzyme activity of each triple co-transformant across individual L-Arabinose concentrations were used. Statistical significance was determined using the Holm–Sidak method, and *P<0.05 was considered significant. (ii) Western blot (seeSupplementary Fig. 3a) ofE. coliwhole-cell lysates to analyse the expression of M5 protein induction with increasing concentrations (corresponding to the concentrations displayed onxaxis of the graph) of L-arabinose. Figure 2: Disruption of ICAM-1 271 dimerization by M5. ( a ) Bacterial two-hybrid assay to assess structural fidelity of ICAM-1 271 and its domains. (i) X-gal indicator plate. All streaks are labelled to represent genes cloned in pTRGnn/pBTnn. (ii) Liquid β-galactosidase assay to measure relative enzyme activity (M.U.) of co-transformant pairs: ICAM-1 271 pTRGnn versus ICAM-1 271 pBTnn (75.16±1.519); ICAM-1 EC pTRGnn versus ICAM-1 EC pBTnn (61.28±6.111); ICAM-1 TM+Cyto pTRGnn versus ICAM-1 TM+Cyto pBTnn (45.45±3.041); ICAM-1 Cyto pTRGnn versus ICAM-1 Cyto pBTnn (10.77±5.195); positive control—CFP10pTRGnn versus ESAT6pBTnn (92.19±4.195); negative control—ICAM-1 EC pTRGnn versus empty pBTnn (2.249±1.189). The graph is the average of three independent assays and s.d. is represented by error bars. All values were tested for significance using a two-tailed unpaired t -test with Welch’s correction. ** P <0.01, **** P <0.0001. ( b ) Bacterial three-hybrid X-Gal indicator plate (i) without L-Arabinose and (ii) with L-Arabinose. Test streaks: triple co-transformant containing ICAM-1 271 pTRGnn, ICAM-1 271 pBTnn and M5pMTSA; control streaks : triple co-transformant containing ICAM-1 271 pTRGnn, ICAM-1 271 pBTnn and empty pMTSA. ( c ) L-Arabinose gradient liquid β-galactosidase assay. (i) Relative β-galactosidase activity (M.U.) of the triple co-transformants ICAM-1 271 pTRGnn/ICAM-1 271 pBTnn versus empty pMTSA (red line) and ICAM-1 271 pTRGnn/ICAM-1 271 pBTnn versus M5pMTSA (black line), is plotted against a range of L-Arabinose concentrations. The graph is the average of three independent assays and s.d. is represented as error bars. Multiple unpaired t -tests to compare enzyme activity of each triple co-transformant across individual L-Arabinose concentrations were used. Statistical significance was determined using the Holm–Sidak method, and * P <0.05 was considered significant. (ii) Western blot (see Supplementary Fig. 3a ) of E. coli whole-cell lysates to analyse the expression of M5 protein induction with increasing concentrations (corresponding to the concentrations displayed on x axis of the graph) of L-arabinose. Full size image M5 interacts with ICAMs Protein–protein interactions between M5 and ICAM-1 or ICAM-4 were evaluated using recombinant proteins. Recombinant ICAM-1 and ICAM-4 were acquired commercially from Sino Biological Inc., China. His-tagged M5 (M5-His) was purified from E. coli BL21 (DE3) strain under denaturing conditions, and the 11-kDa M5 protein dialysed against decreasing concentrations of denaturant ( Fig. 3a ). Because M5 has no homology to any known protein, we deciphered its secondary structural elements by circular dichroism (CD) spectroscopy. The CD spectra of the protein at varying concentrations were analysed using the K 2 D 3 server ( http://k2d3.ogic.ca ) [34] and found to show ~50% β-sheet and ~4% α-helical folds ( Supplementary Fig. 3b–d ). 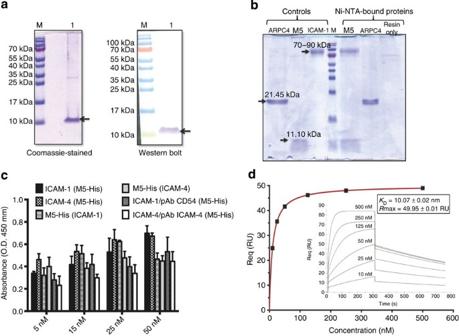Figure 3:In vitroprotein–protein interaction between M5 and ICAMs. (a) Purification of M5-His under denaturing conditions on a Ni-NTA column. Coomassie-stained 10% Tris-Tricine polyacrylamide gel. Western blot of purified M5-His using anti-His antibody.Lane M: Pre-stained protein marker;Lane 2: purified C-terminal His-tagged M5 protein (11.105 kDa). (b)In vitropull-down assay of purified ICAM-1 using M5-His-bound Ni-NTA resin. Coomassie -stained 15% SDS–PAGE.Controls—ARPC4 (nonspecific his-tagged protein; 21.45 kDa); M5-His (11.105 kDa); recombinant ICAM-1 (~90 kDa) are indicated with arrows.Lane M: pre-stained protein marker;Ni-NTA resin pull-down lanes—ICAM-1 pull downs with: M5-His; ARPC4; unbound Ni-NTA resin. (c) ELISA-based analysis of interaction between M5 and ICAM-1 or ICAM-4. M5, ICAM-1 and ICAM-4 were coated at concentrations of 5, 15, 25 and 50 nM. In a subset of wells, ICAM-1- and ICAM-4-coated wells were incubated with anti-ICAM-1 or anti-ICAM-4 antibody, respectively. The overlaid interacting protein is indicated within the parentheses in the graph legend. Subset in which a polyclonal antibody was added before M5 is indicated in the legend. Absorbance by control proteins is shown inSupplementary Fig. 4c. The ELISA for all interactions was performed in triplicates. Histograms of the mean absorbance at 450 nm with s.d. are plotted for each concentration. (d) Kinetic analysis of M5 and human ICAM-4 interaction. Nonlinear regression curve fit forReqplotted against injected ICAM-4 concentrations. Thekaandkdof the interaction were 9.96 × 10−4and 1 × 10−3M, respectively; the derivedKD=10.07±0.02 nM andRmax=49.95±0.23. The inset shows the SPR sensograms of injected ICAM-4 at 20 μl min over immobilized M5 in a CM5 sensor chip. TheReqfor each concentration was calculated after analysis of the association and dissociation from a 1:1 binding model (black lines). The analyte concentration for each sensogram is indicated. Figure 3: In vitro protein–protein interaction between M5 and ICAMs. ( a ) Purification of M5-His under denaturing conditions on a Ni-NTA column. Coomassie-stained 10% Tris-Tricine polyacrylamide gel. Western blot of purified M5-His using anti-His antibody. Lane M : Pre-stained protein marker; Lane 2 : purified C-terminal His-tagged M5 protein (11.105 kDa). ( b ) In vitro pull-down assay of purified ICAM-1 using M5-His-bound Ni-NTA resin. Coomassie -stained 15% SDS–PAGE. Controls —ARPC4 (nonspecific his-tagged protein; 21.45 kDa); M5-His (11.105 kDa); recombinant ICAM-1 (~90 kDa) are indicated with arrows. Lane M : pre-stained protein marker; Ni-NTA resin pull-down lanes —ICAM-1 pull downs with: M5-His; ARPC4; unbound Ni-NTA resin. ( c ) ELISA-based analysis of interaction between M5 and ICAM-1 or ICAM-4. M5, ICAM-1 and ICAM-4 were coated at concentrations of 5, 15, 25 and 50 nM. In a subset of wells, ICAM-1- and ICAM-4-coated wells were incubated with anti-ICAM-1 or anti-ICAM-4 antibody, respectively. The overlaid interacting protein is indicated within the parentheses in the graph legend. Subset in which a polyclonal antibody was added before M5 is indicated in the legend. Absorbance by control proteins is shown in Supplementary Fig. 4c . The ELISA for all interactions was performed in triplicates. Histograms of the mean absorbance at 450 nm with s.d. are plotted for each concentration. ( d ) Kinetic analysis of M5 and human ICAM-4 interaction. Nonlinear regression curve fit for R eq plotted against injected ICAM-4 concentrations. The k a and k d of the interaction were 9.96 × 10 −4 and 1 × 10 −3 M, respectively; the derived K D =10.07±0.02 nM and R max=49.95±0.23. The inset shows the SPR sensograms of injected ICAM-4 at 20 μl min over immobilized M5 in a CM5 sensor chip. The R eq for each concentration was calculated after analysis of the association and dissociation from a 1:1 binding model (black lines). The analyte concentration for each sensogram is indicated. Full size image An in vitro pull-down assay was performed to confirm the interaction between M5 and recombinant ICAM-1. For the interaction analysis, M5-His and a nonspecific histidine-tagged protein Actin-related protein 2/3 subunit 4 (ARPC4, a 22-kDa subunit of the human Arp2/3 protein complex) were immobilized separately on Ni-NTA resin. Recombinant ICAM-1 protein was incubated with M5 or ARPC4-bound resins and the bound proteins eluted subsequently by boiling the resin with 5 × SDS-loading dye. The eluted fractions were analysed by SDS–PAGE and M5-bound Ni-NTA resin was able to retain ICAM-1 ( Fig. 3b ), while the nonspecific protein ARPC4 immobilized on the Ni-NTA column failed to bind ICAM-1. The interactions between M5 and recombinant full-length ICAM-1 or ICAM-4 were also confirmed by reciprocal ELISA-based interaction assays. Unlike ICAM-1, which is constitutively expressed on a variety of cell types, ICAM-4 is expressed exclusively on RBC surface. The homology between ICAM-1 and ICAM-4 Ig-like domains is >40–50% ( www.ebi.ac.uk/Tools/msa/clustalo/ ; Supplementary Fig. 4a,b ). For the assay, M5, ICAM-1 or ICAM-4 proteins were immobilized in ELISA plates and the wells overlaid with the corresponding interacting proteins. After rigorous washing, antibodies against the overlaid proteins were used to detect successful binding. The binding of M5 with ICAM-1 or ICAM-4 was found to be concentration-dependent. A set of wells coated with ICAM-1 and ICAM-4 were also incubated with polyclonal anti-ICAM-1 and anti-ICAM-4 antibodies, respectively, to investigate whether the antibodies would perturb/mask ICAM/M5 interactions ( Fig. 3c ). Binding between ICAMs and M5 was similar to control proteins detected by their specific antibodies (anti-His, anti-ICAM-1 or anti-ICAM-4). These were also specific as neither ICAM-1 nor ICAM-4 interacted with a nonspecific His-tagged protein ARPC4. The controls for the ELISA-based interaction assay are shown in Supplementary Fig. 4c . The M5/ICAM-4 interaction was further studied using surface plasmon resonance (SPR). Using this approach, we found that M5 displayed a strong interaction with ICAM-4 with an equilibrium dissociation constant ( K D )≈10.07±0.02 nM ( Fig. 3d ) and an R max≈49.95±0.23 response unit. The K D and R max were derived using a nonlinear curve-fitting algorithm, calculated based on a one-site-specific binding model (1:1 interaction) using the equation Y = R max × X /( K D + X ), where Y is the SPR equilibrium resonance unit value ( R eq ) and X is the concentration of the injected analyte. A good curve-fit with R 2 equal to 0.9999 was observed using the described parameters. The potent ability of M5 to bind ICAM-1 and ICAM-4 prompted us to evaluate its potential as a modulator of ICAMs, and thereby also assess their role in Mtb and P. falciparum invasion of host cells. ICAM-1 is crucial for M. tuberculosis infection Before investigating whether M5/ICAM-1 interaction had any modulatory effect on Mtb infection, it was prudent to assess whether M5 localized to the ICAM-1 sites on the macrophage cell surface. A localization experiment was performed wherein untreated, anti-ICAM-1 pAb-treated and A205804—a commercial small molecule-selective inhibitor of cellular ICAM-1 expression [35] —treated THP-1 macrophages were incubated with M5, followed by the addition of the cross-linker dimethyl suberimidate. Anti-His, anti-ICAM-1 monoclonal antibody (mAb) and fluorochrome-conjugated secondary antibodies, namely, Alexa Fluor 594 and Alexa Fluor 488, were used for detection of M5 and ICAM-1, respectively ( Fig. 4a , control). Considerable co-localization between M5 and ICAM-1 on untreated THP-1 macrophages was found (Pearson’s coefficient 0.78). Remarkably, A205804-treated macrophages did not stain positive for M5-His on cell surface ( Fig. 4a , A205804-treated), suggesting that the interaction between ICAM-1 and M5 is specific. Anti-ICAM-1 pAb, however, failed to mask ICAM-1 and abrogate M5 binding to the cell surface ( Fig. 4a , antibody-treated). 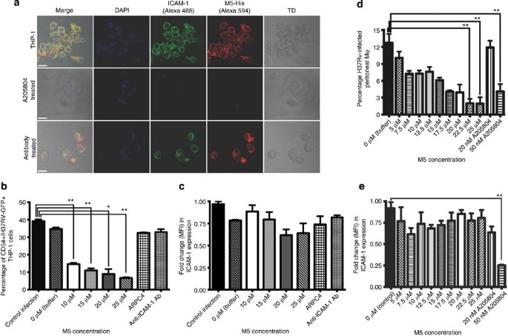Figure 4: Role of ICAM-1 in Mtb infection of activated THP-1 cells. (a) Co-localization of M5-His to sites of ICAM-1 expression on the THP-1 surface. Activated THP-1 cells were incubated with 25 μM M5-His (control) for 1 h and 50 nM A205804 (A205804-treated) or polyclonal anti-ICAM-1 antibody (antibody-treated) for 24 h. A205804- and antibody-treated samples were further incubated with M5-His for 1 h. Co-localization was detected with anti-his and anti-ICAM-1 antibodies. The cells were stained with fluorochrome-conjugated secondary bodies against His-tag (red), ICAM-1 (green) and counterstained with DAPI. Analysis of the co-localization threshold scatter (488 versus 594 nm) was used to determine Pearson’s coefficients: control—0.78, Ab-treated—0.64. Scale bar 20 μm. (b) Bar graph showing the percentages of H37Rv-GFP-infected CD54+ THP-1 macrophages when treated with increasing concentrations of M5 protein (0–25 μM). The data are representative of three independent experiments. Untreated THP-1 macrophages infected with H37Rv-GFP were considered as the positive control against which inhibition of infection was compared for significance. Differences in infection were calculated using unpairedt-tests with Welch’s correction. *P<0.01, **P<0.001. (c) ICAM-1 expression level of untreated and M5-treated THP-1 macrophages using anti-ICAM-1 antibody following infection. The data are represented as fold change in the MFI. The dot plots with gated populations are shown inSupplementary Fig. 5. (d) Percentages of H37Rv-GFP-infected murine peritoneal macrophages when treated with increasing concentrations of M5 protein (0–25 μM). Untreated peritoneal macrophages infected with H37Rv-GFP were considered as the positive control against which inhibition in infection was compared for significance. The data are representative of three independent experiments. Differences in infection were calculated using unpairedt-tests with Welch’s correction. **P<0.001. (e) ICAM-1 expression level of untreated, M5-treated or A205804-treated macrophages using anti-ICAM-1 antibody following infection. The data are represented as fold change in the MFI. Differences in ICAM-1 expression were calculated using unpairedt-tests with Welch's correction. **P<0.001. The dot plots with gated populations are shown inSupplementary Fig. 7a,b. Figure 4: Role of ICAM-1 in Mtb infection of activated THP-1 cells. ( a ) Co-localization of M5-His to sites of ICAM-1 expression on the THP-1 surface. Activated THP-1 cells were incubated with 25 μM M5-His (control) for 1 h and 50 nM A205804 (A205804-treated) or polyclonal anti-ICAM-1 antibody (antibody-treated) for 24 h. A205804- and antibody-treated samples were further incubated with M5-His for 1 h. Co-localization was detected with anti-his and anti-ICAM-1 antibodies. The cells were stained with fluorochrome-conjugated secondary bodies against His-tag (red), ICAM-1 (green) and counterstained with DAPI. Analysis of the co-localization threshold scatter (488 versus 594 nm) was used to determine Pearson’s coefficients: control—0.78, Ab-treated—0.64. Scale bar 20 μm. ( b ) Bar graph showing the percentages of H37Rv-GFP-infected CD54+ THP-1 macrophages when treated with increasing concentrations of M5 protein (0–25 μM). The data are representative of three independent experiments. Untreated THP-1 macrophages infected with H37Rv-GFP were considered as the positive control against which inhibition of infection was compared for significance. Differences in infection were calculated using unpaired t -tests with Welch’s correction. * P <0.01, ** P <0.001. ( c ) ICAM-1 expression level of untreated and M5-treated THP-1 macrophages using anti-ICAM-1 antibody following infection. The data are represented as fold change in the MFI. The dot plots with gated populations are shown in Supplementary Fig. 5 . ( d ) Percentages of H37Rv-GFP-infected murine peritoneal macrophages when treated with increasing concentrations of M5 protein (0–25 μM). Untreated peritoneal macrophages infected with H37Rv-GFP were considered as the positive control against which inhibition in infection was compared for significance. The data are representative of three independent experiments. Differences in infection were calculated using unpaired t -tests with Welch’s correction. **P<0.001. ( e ) ICAM-1 expression level of untreated, M5-treated or A205804-treated macrophages using anti-ICAM-1 antibody following infection. The data are represented as fold change in the MFI. Differences in ICAM-1 expression were calculated using unpaired t -tests with Welch's correction. ** P <0.001. The dot plots with gated populations are shown in Supplementary Fig. 7a,b . Full size image To evaluate the role of ICAM-1 in the uptake of Mtb, phorbol 12-myristate 13-acetate (PMA)-activated THP-1 cells were incubated with M5 at varying concentrations (0–25 μM). In control experiments, a similar number of THP-1 macrophages were treated with buffer solution without any protein/polypeptide as well as with a nonspecific protein ARPC4. The treated cells were infected with Mtb H37Rv-GFP (green fluorescent protein) [36] and infection was monitored by detecting GFP fluorescence through flow cytometry. The treated cells were also analysed for the expression of ICAM-1 by using Alexa Fluor 647-conjugated anti-ICAM-1 antibody. M5-treated cells showed a significant decrease in Mtb infection compared with ARPC4- or buffer-treated THP-1 cells ( Fig. 4b and Supplementary Fig. 5 ). All samples, including those treated with M5, showed a comparable expression level of cell surface ICAM-1 ( Fig. 4c and Supplementary Fig. 5 ). The experiment was performed in triplicates, and was reproducible across each individual repetition. To rule out the possibility that the decrease in Mtb infection in M5-treated cells was because of cell death caused by the protein itself, a viability assay was performed. Treated and untreated THP-1 macrophages were stained with 7AAD, followed by flow cytometry analysis. No change in the cell viability was observed in the M5-treated cells ( Supplementary Fig. 6 ). To study the importance of ICAM-1 in Mtb infection, THP-1 cells were treated with A205804. The reported IC 50 of A205804 for selective inhibition of ICAM-1 is 25 nM [37] . THP-1 macrophages treated with suboptimal (20 nM) and optimal (50 nM) of A205804 were analysed for H37Rv-GFP infection and ICAM-1 expression. The results showed a drastic decrease in Mtb infection in A205804 (50 nM)-treated cells and a concomitant significant drop in ICAM-1 expression ( Fig. 5a,b and Supplementary Fig. 8a,b ). Together, these results suggested a role of ICAM-1 in Mtb infection of mammalian cells. 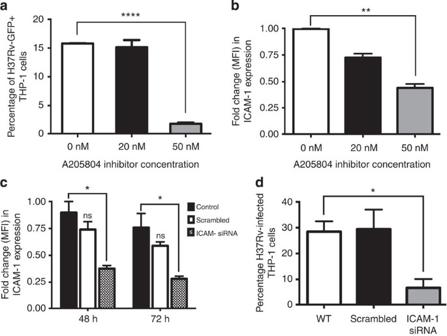Figure 5: ICAM-1 is important for Mtb infection. (a) Percentages of H37Rv-GFP-infected THP-1 cells when treated with suboptimal (20 nM) and optimal (IC5050 nM) A205804. (b) ICAM-1 (CD54) expression level for A205804-treated THP-1 cells. The data are represented as fold change in MFI. Flow cytometry plots for these data are shown inSupplementary Fig. 8a,b. Differences in infection or ICAM-1 expression were calculated using unpairedt-tests with Welch's correction. **P<0.005, ****P<0.0001. (c) ICAM-1 expression in THP-1 macrophages following silencing with 60 nM ICAM-1 siRNA, at 48 and 72 h. Scrambled version of ICAM-1 siRNA was used to validate silencing. The data are represented as fold change in MFI. Flow cytometry dot plots and western blot for ICAM-1 expression is provided inSupplementary Fig. 9a,b. (d) Comparison in percentages of H37Rv-GFP-infected wild-type (WT), scrambled and siRNA-treated THP-1 macrophages. Flow cytometry plots for these data are shown inSupplementary Fig. 9c. All data sets were acquired over three independent experiments. Statistically significant differences in infection were calculated using unpairedt-tests using Welch’s correction. *P<0.05, ns=not statistically significant. Figure 5: ICAM-1 is important for Mtb infection. ( a ) Percentages of H37Rv-GFP-infected THP-1 cells when treated with suboptimal (20 nM) and optimal (IC 50 50 nM) A205804. ( b ) ICAM-1 (CD54) expression level for A205804-treated THP-1 cells. The data are represented as fold change in MFI. Flow cytometry plots for these data are shown in Supplementary Fig. 8a,b . Differences in infection or ICAM-1 expression were calculated using unpaired t -tests with Welch's correction. ** P <0.005, **** P <0.0001. ( c ) ICAM-1 expression in THP-1 macrophages following silencing with 60 nM ICAM-1 siRNA, at 48 and 72 h. Scrambled version of ICAM-1 siRNA was used to validate silencing. The data are represented as fold change in MFI. Flow cytometry dot plots and western blot for ICAM-1 expression is provided in Supplementary Fig. 9a,b . ( d ) Comparison in percentages of H37Rv-GFP-infected wild-type (WT), scrambled and siRNA-treated THP-1 macrophages. Flow cytometry plots for these data are shown in Supplementary Fig. 9c . All data sets were acquired over three independent experiments. Statistically significant differences in infection were calculated using unpaired t -tests using Welch’s correction. * P <0.05, ns=not statistically significant. Full size image To extend the results established in THP-1 macrophages, a similar experiment was performed with murine peritoneal macrophages. BALB/c mice were administered peritoneal injections of thioglycollate. Macrophages from the killed mice were harvested by peritoneal lavage and were enriched overnight to facilitate binding of activated macrophages to assay plates. Following enrichment, the cells were treated with varying concentrations of M5 or A205804 before Mtb H37Rv-GFP infection. We found a dose-dependent reduction in percentages of Mtb-infected macrophages with increasing concentrations of M5 (0–25 μM; Fig. 4d and Supplementary Fig. 7 ). All samples displayed comparable ICAM-1 expression, with the exception of A205804-treated (50 nM) macrophages ( Fig. 4e ). Finally, in an effort to establish the proof-of-concept that ICAM-1 is indeed crucial for Mtb invasion, and could therefore serve as a potential drug target, ICAM-1 expression in THP-1 macrophages was knocked down by siRNA directed against ICAM-1. A series of transfection experiments were set up varying the ratio of transfection agent versus siRNA, and silencing was monitored using western blots and flow cytometry. Maximum silencing was achieved with 60 nM of siRNA pool (Silencer Select, Ambion) at 72 h ( Fig. 5c and Supplementary Fig. 9a,b ). Wild-type, control siRNA (scrambled) and siRNA-transfected THP-1 macrophages were infected with Mtb H37Rv-GFP. We found as much as 70% reduction in infection in the specific siRNA-transfected THP-1 subset ( Fig. 5d and Supplementary Fig. 9c ), while THP-1 macrophages transfected with scrambled siRNA or with transfection reagent alone did now show any reduction in H37Rv-GFP infection. ICAM-4 essential for P. falciparum invasion of erythrocytes Among the many ICAMs identified thus far, ICAM-4 remains an erythrocyte-specific adhesion molecule. Before evaluating the effect of M5 in the invasion of merozoites, we assessed whether M5 binds to ICAM-4 expressed on RBC surface ( Supplementary Fig. 10a ). Co-localization of M5 to the sites of ICAM-4 expression on the RBC surface was performed using anti-His antibody for the detection of M5 and polyclonal anti-ICAM-4 antibody (clone C-20) to probe ICAM-4 on RBC surface. Results showed considerable expression of ICAM-4 on the RBC surface and a robust co-localization (Pearson’s coefficient 0.7) with M5 ( Fig. 6a ). As with ICAM-1 in case of THP-1 macrophages, polyclonal anti-ICAM-4 antibody was also unable to mask the interaction between M5 and ICAM-4 on RBCs ( Supplementary Fig. 10b ). On the basis of these observations, in vitro P. falciparum invasion inhibition assays were performed. Purified mature schizont stage parasites (3D7 strain) were incubated with varying concentrations (7.5–25 μM) of M5 protein. Parasitaemia in control and treated cultures was estimated after 24 h using flow cytometry. A dose-dependent decrease in parasitaemia was observed in M5-treated cultures, with a maximum of ~80% decrease in parasitaemia observed in cultures treated with 25 μM of M5 when compared with untreated cultures ( Fig. 6b ). The result was reproducible over three independent experiments each carried out in duplicate. A similar dose-dependent decrease in parasitaemia was witnessed with three other strains of P. falciparum : Dd2, MCamp (sialic acid-dependent strains) and HB3 (sialic acid-independent strain) upon treatment with M5 ( Fig. 6b ). Further, we assessed the ability of M5 to inhibit invasion in neuraminidase-treated RBCs, as neuraminidase treatment blocks the invasion in sialic acid-dependent strains. Similar level of invasion inhibition was observed in the presence of M5 protein in neuraminidase-treated or -untreated RBCs ( Supplementary Fig. 10c ). Microscopic analysis of Giemsa- and 4',6-diamidino-2-phenylindole (DAPI)-stained culture smears showed that, while new rings were observed in control cultures, M5-treated cultures showed a significantly lesser number of new rings and higher number of free and attached merozoites to RBCs ( Fig. 6c , Supplementary Fig. 10d ). 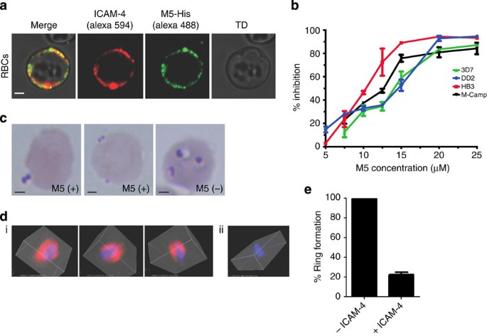Figure 6: Erythrocytic ICAM-4 is involved in merozoite invasion. (a) Co-localization of M5-His to sites of ICAM-4 expression on the RBC surface. Human erythrocytes were incubated with 25 μM recombinant M5-His for 30 min followed by incubation with anti-His and anti-ICAM-4 antibodies. The cells were stained with fluorochrome-conjugated secondary antibodies against His-tag (green) and ICAM-4 (red) followed by confocal microscopy. In a similar experiment, anti-ICAM-4 antibody-treated RBCs were incubated with 25 μM M5-His to detect whether the antibody could mask this interaction (these co-localization results are provided inSupplementary Fig. 10b) Scale bar 2 μm. (b) Invasion inhibition ofP. falciparumstrains 3D7, Dd2, HB3 and MCamp by M5. Purified recombinant M5 protein (7.5–25 μM) was added to mature schizont stage parasite culture and the parasitaemia estimated after 24 h using flow cytometry. The data represent an average of three independent experiments each performed in duplicate. Invasion observed in control culture was taken as 100%. The M5 buffer components did not affect parasite invasion. (c) Giemsa-stained smears of parasite culture treated with M5 at the schizont stage. While new rings were observed in untreated culture (M5(−)), considerable number of free merozoites and merozoites attached to the RBC surface were seen in M5-treated cells (M5(+)). Scale bar 2 μm. All experiments were performed in triplicates for each concentration of M5 and error bars represent s.d. (d) Binding of ICAM-4 on the merozoite surface. (i) Merozoites were incubated with recombinant ICAM-4 protein (175 nM) followed by staining with anti-ICAM-4 antibody and DAPI. (ii) Merozoite in the absence of ICAM-4. (e) Recombinant ICAM-4 protein blocks invasion of human erythrocytes by merozoites. Percoll-purified schizont stageP. falciparumculture was treated with purified ICAM-4 protein. New ring formation was estimated after 15 h using Giemsa-stained smears. Approximately 80% drop in ring formation was observed in ICAM-4-treated culture. Figure 6: Erythrocytic ICAM-4 is involved in merozoite invasion. ( a ) Co-localization of M5-His to sites of ICAM-4 expression on the RBC surface. Human erythrocytes were incubated with 25 μM recombinant M5-His for 30 min followed by incubation with anti-His and anti-ICAM-4 antibodies. The cells were stained with fluorochrome-conjugated secondary antibodies against His-tag (green) and ICAM-4 (red) followed by confocal microscopy. In a similar experiment, anti-ICAM-4 antibody-treated RBCs were incubated with 25 μM M5-His to detect whether the antibody could mask this interaction (these co-localization results are provided in Supplementary Fig. 10b ) Scale bar 2 μm. ( b ) Invasion inhibition of P. falciparum strains 3D7, Dd2, HB3 and MCamp by M5. Purified recombinant M5 protein (7.5–25 μM) was added to mature schizont stage parasite culture and the parasitaemia estimated after 24 h using flow cytometry. The data represent an average of three independent experiments each performed in duplicate. Invasion observed in control culture was taken as 100%. The M5 buffer components did not affect parasite invasion. ( c ) Giemsa-stained smears of parasite culture treated with M5 at the schizont stage. While new rings were observed in untreated culture (M5(−)), considerable number of free merozoites and merozoites attached to the RBC surface were seen in M5-treated cells (M5(+)). Scale bar 2 μm. All experiments were performed in triplicates for each concentration of M5 and error bars represent s.d. ( d ) Binding of ICAM-4 on the merozoite surface. (i) Merozoites were incubated with recombinant ICAM-4 protein (175 nM) followed by staining with anti-ICAM-4 antibody and DAPI. (ii) Merozoite in the absence of ICAM-4. ( e ) Recombinant ICAM-4 protein blocks invasion of human erythrocytes by merozoites. Percoll-purified schizont stage P. falciparum culture was treated with purified ICAM-4 protein. New ring formation was estimated after 15 h using Giemsa-stained smears. Approximately 80% drop in ring formation was observed in ICAM-4-treated culture. Full size image To evaluate the viability of M5-treated parasites, a wash-off experiment was carried out wherein purified mature schizonts (44 h post infection (hpi)) were incubated with RBCs either in presence or absence of M5. The schizonts were allowed to rupture and merozoites allowed to invade new RBCs to form ring-stage parasites. In the M5-treated set there was a threefold reduction in RBC invasion by merozoites compared with control. Following initial invasion, M5 was washed off from the cultures and the parasite growth monitored for the next three cycles. There was no difference in the fold change in parasitaemia in control and M5-treated sets in subsequent cycles ( Supplementary Fig. 10e ). To rule out any inhibitory effect of M5 on parasite development, we also assessed parasite growth across asexual stages in presence of M5 protein; the result showed that M5 has no effect on parasite developmental stages ( Supplementary Fig. 10f ). Together, these results suggested that the decrease in parasitaemia observed in M5-treated cultures was because of invasion inhibition and not because of loss of viability of the parasites or any other inhibitory effect of M5 on different stages of parasite development. To establish whether P. falciparum merozoites bind directly to ICAM-4, recombinant ICAM-4 was added to in vitro P. falciparum cultures and the binding detected using anti-ICAM-4 antibody. As shown in Fig. 6d , significant binding of ICAM-4 on the merozoite surface was observed. These results suggest that merozoites express ligand(s) that bind to ICAM-4 present on the RBC surface. Following this, recombinant ICAM-4 (175 nM) was added to the merozoite invasion assay mix and new ring formation monitored. The addition of recombinant ICAM-4 to parasite cultures blocked the invasion of newly released merozoites and in-turn reduced development of ring-stage parasites by 80% when compared with control-untreated cultures ( Fig. 6e ). Together, these results implicate ICAM-4 in the invasion of P. falciparum merozoite into RBCs. ICAM-1 has been classified as a type I transmembrane protein with an extracellular region consisting of 453 amino acids, arranged in the form of five Ig-like domains. ICAM-4, on the other hand, is a relatively small molecule that comprises two Ig-like extracellular domains and is expressed exclusively on RBC surface. Without exception, all ICAMs bind to CD11a/CD18 (LFA-1, α L β 2 ) on leukocytes. ICAM-1, ICAM-2 and ICAM-4 also interact with the granulocyte/monocyte-enriched β 2 integrin CD11b/CD18 (Mac-1, α M β 2 ) [38] , [39] , [40] . ICAM-4 is unique in that it is the only Ig superfamily member that has also been shown to bind to CD11c/CD18, αv integrins (α v β 1 , α v β 3 and α v β 5 ) on nonhaemopoietic cells, α 4 β 1 on haemopoietic cells and α IIb β 3 on platelets [41] , [42] , [43] . However, the role of ICAMs in the invasion by two important intracellular pathogens, Mtb and P. falciparum , was hitherto unknown. While no direct evidence connecting Mtb invasion of host cells and ICAM-1 has thus far come to light, there are studies that show an increase in the expression levels of ICAM-1 on macrophages infected with Mtb [44] . In addition, even though this change in expression could be ascribed as a response of the immune system to recruit more leukocytes to the site of bacterial infection, the increase is so abnormally high [45] that we speculate it to be a pathogen-specific response. In the present study, while screening for host-interacting molecules of Mtb using a human cDNA library, ICAM-1 was identified as the host counterpart involved in separate interactions with C-terminal regions of two mycobacterial metabolic proteins IlvB2 and fadB3 (Rv1715). While there is little literature available on IlvB2, fadB3 has been characterized as a secretory, nonessential protein [46] involved in fatty acid metabolism. In the past two decades bacterial metabolic enzymes have begun to be recognized for their moonlighting capabilities and as determinants of virulence. This has been previously reviewed in detail, with many such proteins now known for Mtb [47] . Interaction with host ICAM-1 indicates possible moonlighting functions of IlvB2 and fadB3 and will require further investigation. To investigate whether host ICAM-1 does indeed play a role in Mtb infection, we screened ICAM-1 against a synthetic polypeptide library and identified an 84-amino-acid-long M5 protein that bound ICAM-1 with high affinity. We have previously used a similar approach to identify synthetic proteins that bind and inhibit crucial enzymes of Mtb [29] . Since ICAM-1 possesses extracellular Ig-like domains, a transmembrane domain and a cytoplasmic domain, a bacterial two-hybrid-based analysis was performed with M5 as a bait, with different domains of ICAMs; ICAM-1 271 , ICAM-1 EC , ICAM-1 TM+Cyto and ICAM-1 Cyto as ligands. The analysis showed that M5 binds primarily to the extracellular domains of ICAM-1 and that this binding also prevents the dimerization of ICAM-1. Interaction between M5 and ICAM-1 was further confirmed using ELISA, co-localization as well as by pull-down assays. Interestingly, SPR experiments also revealed M5 to interact with ICAM-4 with a high affinity, characterized by K D ≈10.07 nM. Surprisingly, addition of anti-ICAM pAbs in the M5-ICAM-binding reactions did not seem to diminish M5’s ability to bind ICAM-1 or ICAM-4. This may possibly be because the antibody-binding epitope(s) are distinct from the M5-binding domain. Most notably, a study by Bartholdson et al. [48] also reported that the P. falciparum protein MTRAP (expressed on merozoites and involved in motility and invasion) is a ligand to Semaphorin-7A on RBCs and showed that anti-MTRAP mAb and anti-Semaphorin-7A monoclonal and polyclonal antibodies were unable to block merozoite invasion into RBCs. Having identified a potent ICAM-binding synthetic polypeptide, we next assessed the role of ICAMs in the context of two pathogens, M. tuberculosis and P. falciparum , in host cell invasion. It is well known that Mtb infects alveolar macrophages through a series of events that ultimately determine whether the bacilli is able to evade the innate immune response and successfully survive intracellularly [49] . The uptake itself engages a myriad of phagocytic receptors, thereby initiating specific signalling pathways and modulating several immunobiological processes during and after phagocytosis [50] . Once we identified host ICAM-1 to be possibly implicated in host–pathogen interactions, the effect of M5 on Mtb invasion of macrophages was analysed. The results showed >70% inhibition in Mtb invasion, consistently across THP-1 as well as murine peritoneal macrophages, thereby suggesting the role of ICAM-1 in Mtb entry into the macrophages. To further confirm the role of ICAM-1 as an Mtb receptor, ICAM-1 expression on THP-1 macrophages was blocked by the addition of A205804—whose use as an ICAM-1 expression inhibitor has been described earlier [35] —as well as PMA-activated THP-1 cells using siRNAs. H37Rv infection was inhibited in these treated cells by as much as 70% compared with wild-type and control siRNA-transfected macrophages. Together, the results show that M5 binds ICAM-1 extracellularly, but bears no effect on the host cell ICAM-1 expression. There are previous reports of disruption of the ICAM-1/LFA-1 interaction using mAbs, ICAM-1 or LFA-1 derived peptides as well as other small molecule inhibitors [51] , [52] , [53] , leading to altered immune signalling to control inflammatory and/or autoimmune responses. In case of pathogenic infections, mAb against ICAM-1 as well as soluble ICAM-1 (comprising only the ectodomain) have been previously shown to block Human Rhinovirus infection [54] . While similar blockade by antibodies was absent in case of Mtb, M5 is the first such completely de novo protein binder that blocks Mtb entry to a large extent into host cells. ICAMs have also been implicated in malaria, although only during the process of cytoadherence. P. falciparum -infected erythrocytes sequester in deep vascular beds by binding to ICAM-1 expressed on the surface of endothelial cells [55] . The rationale behind examining the binding of M5 to ICAM-4 and then to study whether it could also modulate P. falciparum infection was threefold. First, all the Ig-like superfamily molecules display a good degree of homology and bind common ligands. ICAM-1 and ICAM-4 further share the ability to also bind Mac-1 (refs 38 , 56 , 57 ). These interactions primarily elicit immunologically important functions of cell adhesion and inflammation. Second, P. falciparum -infected erythrocytes express a protein PfEMP1 (a member of the ‘var’ antigen family) that binds endothelial ICAM-1 and is responsible for the manifestation of complicated cerebral malaria [26] . Finally, very recently, another member of the Ig superfamily, Basigin, has been characterized as a receptor for P. falciparum invasion of erythrocytes [15] . Basigin is an RBC surface molecule expressed as two isoforms; one isoform has two Ig-like domains (much like ICAM-4) and the other isoform has three Ig-like domains. Keeping the above-mentioned studies in mind, while analysing our results in context of M5 to not only bind ICAM-1 but also inhibit intracellular invasion of Mtb by virtue of its interaction, we were curious to explore whether M5 could also bind other ICAMs and elicit similar responses to other pathogens. P. falciparum infection in RBCs provided a unique system for this in that RBCs exclusively express ICAM-4 (and no other ICAMs) on their cell surface. After confirming in vitro interaction between M5 and ICAM-4, and proceeded with assessing its effect on P. falciparum invasion. A significant block (>80%) in parasite invasion was observed in the presence of M5 for both chloroquine-sensitive as well as -resistant lines, suggesting a role of ICAM-4 as a receptor for P. falciparum invasion of RBC. Further, M5 was able to block invasion of both sialic acid-dependent as well as -independent parasite lines. Invasion involves various events between receptors on host RBCs and ligands on the merozoites, the invasive form of the parasite. Microscopic analysis showed that the attachment of merozoites to host blood cells was unaffected, indicating the role of ICAM-4 at later stages of invasion post attachment. In addition, purified recombinant ICAM-4 inhibited merozoite invasion, possibly because recombinant ICAM-4 competed directly with its membrane-bound homologue on the RBC surface. Furthermore, recombinant purified ICAM-4 bound released merozoites, thereby advocating the presence of ligand(s) on the merozoite surface that interact with ICAM-4. Of the various known receptor–ligand interactions, none except Basigin has been shown to be essential across multiple P. falciparum strains, suggesting redundant pathways for invasion. The inhibition of erythrocyte invasion after addition of M5 by multiple P. falciparum strains (3D7, Dd2, MCamp and HB3) suggests that ICAM-4 is a critical host receptor marked for the invasion process. In summary, we describe here a systematic screen of an Mtb genomic library with human host library leading to the identification of ICAM-1 as a host-interacting protein. In addition, we identify a completely de novo protein M5, unearthed from a codon-shuffled peptide library, that acts as a potent binder to ICAM-1 and ICAM-4. Using M5 and a well-known inhibitor of ICAM-1 expression, A205804, as well as siRNA-based knockdown experiments, we further demonstrate ICAMs as receptors essential for entry of two important intracellular pathogens, namely, Mtb and P. falciparum into mammalian cells. This study, we believe, provides two major outcomes. First, it identifies two previously known adhesion molecules, ICAM-1 and ICAM-4, as possible receptors or accessory molecules implicated in host cell invasion by Mtb and P. falciparum . Modulating the two ICAMs provides a proof-of-concept to their potential as new drug targets, with the synthetic polypeptide M5 presenting a template for designing lead peptidomimetic drug(s) or small inhibitors against the two important intracellular pathogens. Second, it also establishes an opportunity of utilizing the described de novo peptide libraries to discover potent binders of previously known drug targets/receptors for other pathogens. Ethics statement BALB/c female mice at 8 weeks of age were used for this study following the institutional ethical committee guidelines. All animal experiments were conducted in accordance with the guidelines approved by the Institutional Animals Ethics Committee of ICGEB, New Delhi, India. Human blood was used for P. falciparum culture in this study. Donor blood was obtained from Rotary blood bank (RBB), New Delhi, India. RBB follows stringent screening procedures, careful documentation and Good Laboratory Practices for collecting, processing and testing blood and is an ISO 9001:2008 certified blood bank established in 2002. Mtb library construction The Mtb H37Rv genomic library and the dicodon library were constructed as described earlier [29] , [33] . Briefly, Mtb H37Rv genomic DNA was isolated from bacteria grown in 7H9 broth supplemented with ADC enrichment as described previously [58] and subjected to partial digestion with Hae III and Nla I. The digested fragments varying from 200 bp to 2 kb in length were eluted from a 1% agarose gel. Annealed phosphorylated (P) and PAGE-purified double-stranded (ds) hairpin (see Supplementary Table 2 ) was ligated to eluted genomic DNA fragments and the ligated products digested with Xba I. The ligated DNA fragments were amplified using primers HP2P, bHP2P and cHP2P (see Supplementary Table 2 ). These primers were designed such that they generated phosphorylated 5′ PCR-amplified fragments in three consecutive frames, which were then cloned into Sna BI-digested and dephosphorylated pBTnn vector. The library DNA was electroporated into XL-1 competent strains and plated on chloramphenicol (30 μg ml −1 )-containing LB agar plates. Dicodon library construction Hundred nanograms of each of the fourteen [28] P-5′ DNA dicodons were taken in a 20-μl ligation reaction containing 7.5% polyethylene glycol and gently heated to 55 °C. The temperature was then slowly brought down to 4 °C. The DC mixture was incubated at 4 °C for 24 h. To this mixture were added 100 pmol of P-5′, PAGE-purified ds hairpins that had been self-annealed earlier. The ligation temperature was increased to 16 °C, and the incubation prolonged for another 12 h. The DNA was precipitated from the ligation mixture and extracted once with phenol/chloroform. The resuspended DNA was digested with Xba I for 4 h at 37 °C, after which 1 μl of the digested DNA was used as a template for PCR using HP2P that served both as a forward and reverse primer. The PCR products were eluted using DEAE membrane and fractionated based on their lengths (50–400 bp). The purified fragments were used directly as inserts for creation of de novo libraries in Sna BI-cut and dephosphorylated pBTnn and pTRGnn vectors. The human lung cDNA library, cloned into the pTRG vector, was acquired commercially from Stratagene, CA, USA. ICAM-1 271 and M5 cloning The 841-bp-long ICAM-1 271 was divided into separate domains, namely, extracellular (EC, 675 bp), transmembrane and cytoplasmic (TM+Cyto, 193 bp) and cytoplasmic tail (Cyto, 112 bp) and each was cloned into Sna BI-cut and dephosphorylated pTRGnn and pBTnn vectors, respectively. The inserts were PCR-amplified using the following primer sets: ICAM-1 271 : ICAM-For, ICAM-Rev; ICAM-1 EC : ICAM-For, ICAM-D3D5-Rev; ICAM-1 TM+Cyto : ICAM-D3D5-For, ICAM-Rev and ICAM-1 Cyto : ICAM-Cyto-For, ICAM-Rev (see Supplementary Table 2 ). The M5-encoding DNA sequence was PCR-amplified using HP2P primer and used as an insert in a blunt-end cloning into Sna BI-cut and dephosphorylated pMTSA vector [33] . The resulting plasmid was used for three-hybrid studies as well as for expression of C-terminal His-tagged M5 protein. Bacterial two-hybrid screen The bacterial two-hybrid experiment was carried out according to the protocol provided by the manufacturer (Stratagene). Briefly, plasmids pBTnn, containing Mtb genomic DNA, and pTRGnn, containing human lung cDNA were used to co-transform R1 reporter cells. The co-transformants were plated on X-Gal indicator plates containing kanamycin (50 μg ml −1 ), chloramphenicol (30 μg ml −1 ), tetracycline (12.5 μg ml −1 ), X-Gal (80 μg ml −1 ), Isopropyl β-D-1-thiogalactopyranoside (25 μM) and phenylethyl-β-D-thiogalactoside (200 μM). Visual blue–white selection on the indicator plates was the initial criteria for screening of colonies. Mycobacterial proteins CFP10 and ESAT6, that are known to form a tight 1:1 complex [32] and have been shown previously to interact using a bacterial two-hybrid system [33] , were cloned into pBTnn and pTRGnn, respectively, and used as positive controls. To discover interacting de novo peptide/polypeptide/protein partners to known proteins, the bacterial two-hybrid experiments between ICAM-1 271 pTRGnn and dicodon libraries cloned in pBTnn were performed as described above. All interacting pairs thus found were retransformed repeatedly, segregated and re-cloned to confirm the interactions. Liquid β-galactosidase assays To confirm and quantify the strength of protein–protein interactions, the expression level of reporter enzyme β-galactosidase was compared with the positive control in a colorimetric enzymatic assay [59] . To ascertain statistical significance, a Student’s t -test was used to compare all values to the negative control. Values of P <0.01 were considered as significant. Bacterial three-hybrid screen ICAM-1 271 and its various fragments ( Fig. 2 ) cloned in both pBTnn and pTRGnn were used to set up bacterial two-hybrid screens. All co-transformants were analysed for the presence of both plasmids by PCR using vector-specific primers. ICAM-1 271 pBTnn/ICAM-1 271 pTRGnn, ICAM-1 EC pBTnn/ICAM-1 EC pTRGnn and ICAM-1 TM+Cyto pBTnn/ICAM-1 TM+Cyto pTRGnn interactions displayed blue colour, while ICAM-1 Cyto pBTnn/ICAM-1 Cyto pTRGnn interaction yielded white colonies. The cells containing the co-transformants were used to make competent cells, which were further transformed with M5pMTSA and plated on X-Gal indicator plates, both in the presence and absence of L-arabinose (1% w/v). The competent cells carrying the two plasmids with ICAM-1 Cyto (that yielded white colonies) and transformed with M5pMTSA were treated as negative control. Transforming ICAM-1 271 carrying competent cells with empty pMTSA served as a vector control. The plates were incubated at 30 °C and reversion of colony colour from blue to white—upon induction of M5 expression by L-arabinose—indicated disruption of ICAM-1 dimerization. The basis and validation of the bacterial three-hybrid system has been described previously [33] . Arabinose gradient liquid β-galactosidase assay A liquid β-galactosidase assay, but with increasing concentrations of L-Arabinose (0.0, 0.005, 0.01, 0.05, 0.1, 0.5, 1.0, 1.5 and 2.0 mM), was carried out in triplicates as described previously [33] . To ascertain statistical significance, a Student’s t -test was used to compare all values to the negative control. Values of P <0.01 were considered as significant. E. coli BL21 (DE3) strain harbouring M5 cloned into pMTSA vector [33] was induced with corresponding concentrations (0.0–2.0 mM as used in liquid β-galactosidase assay) of L-arabinose, and whole-cell lysates of 5 ml cultures were analysed by western blot analysis for the expression of M5-His using anti-His antibody (anti-His mAb, 1 mg ml −1 , 1:3,000 dilution). Expression and purification of recombinant M5 To functionally characterize M5-His, the 11-kDa C-terminal His-tagged polypeptide was overexpressed in a heterologous E. coli expression system through arabinose induction. The expressed protein was found in inclusion bodies. BL21 (DE3) cells carrying M5pMTSA plasmid were inoculated in liquid culture media and grown overnight at 37 °C in the presence of streptomycin (50 μg ml −1 ). After growing the culture to mid-log phase, it was induced with 0.2% L-arabinose at 25 °C for 12 h. The culture was pelleted and washed with 1 × PBS and the cell pellet resuspended in lysis buffer (1 × PBS containing 2 mM phenylmethylsulphonyl fluoride) and sonicated till a clear lysate was obtained. The pellet fraction was resuspended in a buffer containing 25 mM Tris-HCl, 0.3 M NaCl and 8 M urea, and the proteins were extracted using centrifugation. The resultant supernatant was bound to Ni-NTA superflow resin at room temperature. The bound proteins were eluted from Ni-NTA through an imidazole gradient between buffer A (8 M urea, 25 mM Tris-HCl, 0.3 M NaCl, 20 mM Imidazole, pH 8.5) and buffer B (8 M urea, 25 mM Tris-HCl, 0.3 M NaCl, 500 mM Imidazole, pH 8.5). The purification was performed using an FPLC system (AKTA purifier, GE, USA). The pooled eluant was dialysed against 25 mM Tris-HCl, 0.3 M buffer, pH 8.5, by step-dialysis to achieve gradual removal of urea from 8 to 0 M. The protein was analysed on a Tris-Tricine PAGE and confirmed using western blot using anti-His antibody (Sigma Aldrich, USA; Fig. 3a ). The fractions containing >90% of the recombinant protein were pooled and step-dialysed against decreasing urea concentrations until the denaturant had been completely removed. The purified protein was analysed on Tris-Tricine PAGE and was found to be >90% pure. CD spectroscopy suggested M5 to be composed of ~50% β-sheets ( Supplementary Fig. 3b ). The secondary structure spectral analysis was carried out using the K 2 d 3 server ( http://k2d3.ogic.ca ) [60] . In vitro protein interaction assays Recombinant ICAM-1 (Cat. no. 10346-HCCH-100) and recombinant ICAM-4 (Cat. no. 13327-H02H-100) were acquired from Sino Biological, China. Interactions between M5-His and recombinant ICAMs were ascertained by various in vitro protein techniques described below. In vitro protein pull-down M5-His (10 μg) was bound to the Ni-NTA resin. Beads were washed twice with wash buffer I (25 mM Tris-HCl, 0.3 M NaCl, pH 8.5), and once with wash buffer II (1 × PBS, 0.1% Tween-20, 14 mM β-ME). Beads were then blocked with 1% polyvinylpyrrolidone for 1 h. Following this, 10 μg of ICAM-1 was added and the constituents incubated at room temperature for 2 h. In a control experiment, Ni-NTA beads were blocked with 1% polyvinylpyrrolidone and incubated with 10 μg of ICAM-1 protein at room temperature for 2 h. Finally, beads were washed extensively with wash buffer I. Resin-bound proteins were eluted by boiling beads in 5 × SDS-loading dye and analysed by 15% SDS–PAGE. ELISA-based protein interaction ELISA-based detection of in vitro protein–protein interaction was carried out as reported earlier, with slight modifications in the protocol [61] . Briefly, purified proteins were coated on a 96-well ELISA plate (NuncMaxisorb ELISA plates) at varying concentrations (25, 50, 75 and 100 ng) in 0.1 M carbonate/bicarbonate-coating buffer, pH 9.6. The protein-coated plates were blocked with blocking buffer containing 1 × PBS, 0.1% Tween-20 and 1% BSA, at room temperature for 2 h. Subsequently, the plates were washed three times with PBST (1 × PBS, 0.1% Tween-20). The washed plates were incubated with a 1:1 ratio of the interacting protein partner in dilution buffer (1 × PBST containing 0.5% BSA), for 1 h at room temperature. Only the test wells were incubated with the interacting protein partner while the control wells were incubated with a noninteracting protein. Following washing, primary antibody (anti-his mAb—1 mg ml −1 , 1:3,000 dilution; anti-ICAM-1 pAb—200 μg ml −1 , 1:500 dilution; anti-ICAM-4 pAb—200 μg ml −1 , 1:500 dilution, see Supplementary Table 1 ) against the overlaid protein was added to corresponding test and control wells and incubated for 1 h at room temperature with gentle shaking. The horseradish peroxidase-conjugated 2° antibody (0.8 mg ml −1 , 1:5,000 dilution) was added to the washed plates and samples incubated at room temperature for 1 h with gentle shaking. The ELISA plates were thoroughly washed again, followed by addition of soluble TMB substrate. The plates were incubated at 37 °C for 30 min and the reaction stopped by addition of 1 N H 2 SO 4 . Absorbance was measured at 450 nm using a plate reader. Surface plasmon resonance SPR assays were performed on BIACORE 2000 instrument (GE Healthcare) at 37 °C, using HBS-EP buffer (general purpose buffer, degassed and ready to use 0.01 M HEPES pH 7.4, 0.15 M NaCl, 3 mM EDTA, 0.005% v/v Surfactant P20; GE Healthcare). M5-His was immobilized up to 50 response units in a flow cell of CM5 sensor-chip (GE Healthcare). For kinetic measurements, increasing concentrations of recombinant ICAM-4 were injected over immobilized M5-His as well as the reference flow cell, at a flow rate of 20 μl min −1 . The surfaces were regenerated with a pulse of 10 mM Glycine at pH 1.5 at the end of each injection cycle. Duplicate injections of the same concentration in each experiment were superimposable, demonstrating no loss of activity after surface regeneration. Reference-subtracted sensorgrams were analysed using the Biacore evaluation software 4.1.1 (GE Healthcare). To determine the kinetic parameters of the interaction, binding responses in the steady-state region of the sensorgrams were plotted against analyte concentration and fitted to the standard 1:1 (Langmuir) bimolecular interaction with simultaneous fitting of k a and k d . Kinetic constants were calculated by nonlinear regression fitting to the association and dissociation phases of the sensorgrams. H37Rv infection of macrophages THP-1 cells were propagated in RPMI-1640 medium with 2 mM L-Glutamine (Gibco, Life Technologies) supplemented with 10% FBS, 50 μg ml −1 cefotaxime (Amresco LLC, USA) and 0.250 μg ml −1 amphotericin B (Amresco LLC; hereafter referred to as ‘complete media’). In all, 1 × 10 6 cells were seeded in a 12-well plate and activated with PMA. Forty-eight hours later, cells were incubated overnight with complete media containing varying amounts of M5-His, nonspecific protein (ARPC4-His, 10 μM), polyclonal anti-ICAM-1 antibody (Santa Cruz Biotechnology, USA, Clone H-108) and ICAM-1 inhibitor A205804 {(4-[(4-Methylphenyl) thio]thieno [2,3-c]pyridine-2-carboxamide), (Tocris Bioscience, R&D Systems, UK)}, in triplicates along with appropriate cell controls. The cells were infected with Mtb H37Rv-GFP (see Supplementary Table 1 ) at an multiplicity of infection of 10 and incubated at 37 °C and 5% CO 2 for 4 h after which the cells were scraped from the wells. The pelleted cells were washed once with 1 × PBS followed by a wash with FACS wash buffer (1 × PBS, 3% FBS). The cells were then incubated for 1 h with Alexa Fluor-conjugated anti-ICAM-1 mAb (Santa Cruz Biotechnology, Clone 15.2). Fixed cells (4% paraformaldehyde) were subjected to flow cytometry analyses on the BD FACSCanto II platform. Fluorescence signals were detected with both FL1 (excitation 488, filter 530/30) and FL4 (excitation 640, filter 660/20) channel and analysed based on emission spectra. Five 8-week-old female BALB/c mice were administered 2 ml of thioglycollate through the intraperitoneal route. On the fifth day, mice were killed and immune cells recovered by lavage of the peritoneal cavity. Enrichment of macrophages was carried out by allowing them to settle and attach to the surface of assay wells in the presence of complete media lasting 24 h. Mtb H37Rv-GFP infection assays in the presence of M5 or A205804 inhibitor were performed as described above. ICAM-1 siRNA transfection Pre-validated and inventoried Silencer Select siRNAs against ICAM-1 (Ambion, Life Technologies, see Supplementary Table 2 ) were used to transfect PMA-activated THP-1 cells. Transfections were carried out with DharmaFECT 2 transfection reagent (Dharmacon, GE Lifesciences) following the manufacturer’s protocol. Briefly, 0.5 × 10 6 THP-1 cells were seeded in 12-well plates in complete media in the presence of PMA to trigger activation. Following a media change, the cells were allowed to rest for 24 h. ICAM-1 or scrambled siRNA (60 nM) was used to transfect THP-1 in antibiotic-free RPMI-1640 containing 10% FBS. Silencing of ICAM-1 expression following transfections was monitored at 48 and 72 h by western blot and flow cytometry analyses. The western blots were probed with primary antibodies (anti-ICAM-1 pAb, 200 μg ml −1 , 1:500 dilution; anti-GAPDH, 1 mg ml −1 , 1:5,000 dilution) followed by washing. The blots were incubated with secondary antibody (IRDye 800CW-conjugated, 1 mg ml −1 , 1:15,000 dilution, LI-COR Inc., USA, see Supplementary Table 1 ) for an hour and the signal detected on a LI-COR Odyssey CLx Infrared Imaging System. Maximum silencing was observed at 72 h, at which time point Mtb H37Rv-GFP infection assays were performed as described above. Parasite culture In vitro P. falciparum cultures were maintained following standard protocols reported in ref. 62 . Briefly, the parasite was cultured in O + human erythrocytes in RPMI-1640 medium (Invitrogen) supplemented with 0.5% AlbumaxII, 0.005% (w/v) hypoxanthine, 0.02% (w/v) sodium bicarbonate and 10 μg ml −1 gentamycin at 37 °C. The parasite cultures were synchronized by sorbitol treatment as reported earlier [63] . Staining of receptors and co-localization Human erythrocytes were fixed with 1% paraformaldehyde for 1 h at room temperature (RT). They were washed with 1 × PBS followed by blocking in 3% BSA in 1 × PBS containing 0.2% Tween for 30 min, following which the cells were incubated with anti-ICAM-4 pAb (200 μg ml −1 , 1:200 dilution) in blocking buffer for 1 h at RT. The cells were washed three times with 1 × PBS containing 0.2% Tween-20 followed by incubation with appropriate fluorochrome-conjugated secondary antibody (2 mg ml −1 , 1:1,500 dilution) for 1 h at RT. After washing, the samples were analysed under Nikon A1 confocal microscope. Human erythrocytes were incubated with 25 μM M5 for 1 h. Cells were cross-linked with 50 mM dimethyl suberimidate dihydrochloride in 100 mM sodium borate buffer (pH 9.5) containing 1 mM MgCl 2 for 1 h followed by fixing with 1% paraformaldehyde for 1 h at RT. The reaction was quenched with 0.1 M glycine in 1 × PBS, pH 7.4 for 1 h at RT. The cells were washed with PBS followed by blocking with 3% BSA in 1 × PBS containing 0.2% Tween for 30 min. Cells were incubated with anti-ICAM-4 pAb and anti-His mAb (1 mg ml −1 , 1:1,500) in blocking buffer for 1 h at RT. The cells were washed three times with 1 × PBS containing 0.2% Tween-20 followed by incubation with appropriate fluorochrome-conjugated secondary antibodies (2 mg ml −1 , 1:1,500 dilution, see Supplementary Table 1 ) for 1 h at RT. After washing, the samples were analysed under Nikon A1 confocal microscope. For the antibody-masking experiments, the same protocol was followed but with erythrocytes incubated with anti-ICAM-4 pAb (Santa Cruz Biotechnology, Clone C-20) before addition of M5. THP-1 macrophages were stained similarly, both for surface expression of ICAM-1 as well as co-localization, with the slight modification that macrophages were fixed after incubation with the fluorescent-conjugated secondary antibodies. Invasion inhibition assay The effect of M5 on parasite invasion was evaluated on four different strains of P. falciparum (3D7, Dd2, HB3 and MCamp; see Supplementary Table 1 ). Invasion inhibition assay was performed as described previously [64] . Briefly, the haematocrit and parasitaemia of synchronized schizont stage cultures was adjusted to 2% and 1%, respectively. M5 protein (7.5–25 μM) was added to the parasite culture in 96-well plates and parasitaemia estimated after an incubation of 24 h using flow cytometry. Briefly, cells from samples were collected and washed twice with PBS followed by staining with ethidium bromide (10 μg ml −1 ) for 30 min at room temperature in the dark. The cells were subsequently washed twice with PBS and analysed on FACSCalibur (Becton Dickinson) using the CellQuest software. Fluorescence signal (FL2) was detected with the 590-nm band pass filter using an excitation laser of 488 nm collecting 100,000 cells per sample. Uninfected RBCs stained in similar manner were used as background. Following acquisition, data were analysed for % parasitaemia of each sample by determining the proportion of FL2-positive cells using CellQuest. The data represent an average of three independent experiments conducted in duplicate. Merozoite invasion inhibition—staining for microscopy Synchronized P. falciparum culture containing schizonts was percoll-purified. The schizont-enriched culture was grown for 6 h in complete RPMI-1640 medium containing 25 μM purified recombinant M5 protein at 2% haematocrit and 10% parasitaemia in a 12-well plate. The cells were harvested by centrifugation at 4,000 × g. Thin smears were made on glass slides followed by methanol fixation and staining with Giemsa or DAPI. Giemsa-stained slides were analysed on Zeiss AxioCam ERc 5s microscope and DAPI-stained slides on Nikon A1 confocal microscope. Merozoite staining Synchronized P. falciparum culture containing schizonts was percoll-purified. The schizont-enriched culture was grown for 8-10 h in complete RPMI-1640 medium containing purified recombinant ICAM-4 protein. Released merozoites having bound ICAM-4 protein were harvested by centrifugation at 3,300 × g for 5 min. The merozoites were fixed with 1% paraformaldehyde for 1 h at RT, followed by blocking with 3% BSA in PBS for 30 min at RT. After washing with PBS, the merozoites were incubated with anti-ICAM-4 antibody for 1 h at RT followed by incubation with secondary antibody for 1 h at RT. The merozoites were washed and captured on lysine-coated slides followed by analysis under Nikon A1 confocal microscope. Parasite growth inhibition assays To rule out any inhibitory effect of M5 on parasite developmental stages, we assessed the parasite developmental stage profile in the presence of M5 protein. Early ring-stage parasites were incubated with M5 protein (15 μM) and allowed to grow through different developmental stages. For microscopic analysis, smears were made from each well at different time points (10, 20, 24, 30, 36, 48 and 52 hpi), fixed and subsequently stained with Giemsa, and the number of parasites at different developmental stages counted. How to cite this article: Bhalla, K. et al. Host ICAMs play a role in cell invasion by Mycobacterium tuberculosis and Plasmodium falciparum . Nat. Commun. 6:6049 doi: 10.1038/ncomms7049 (2015).